Dimensionality-driven insulator–metal transition in A-site excess non-stoichiometric perovskites Coaxing correlated materials to the proximity of the insulator–metal transition region, where electronic wavefunctions transform from localized to itinerant, is currently the subject of intensive research because of the hopes it raises for technological applications and also for its fundamental scientific significance. In general, this tuning is achieved by either chemical doping to introduce charge carriers, or external stimuli to lower the ratio of Coulomb repulsion to bandwidth. In this study, we combine experiment and theory to show that the transition from well-localized insulating states to metallicity in a Ruddlesden-Popper series, La 0.5 Sr n +1−0.5 Ti n O 3 n +1 , is driven by intercalating an intrinsically insulating SrTiO 3 unit, in structural terms, by dimensionality n . This unconventional strategy, which can be understood upon a complex interplay between electron–phonon coupling and electron correlations, opens up a new avenue to obtain metallicity or even superconductivity in oxide superlattices that are normally expected to be insulators. The fundamental distinction between insulators and metals relies on how electrons behave nearest Fermi level ( E F ), which separates the occupied from unoccupied electron energy levels. For an insulator, the E F lies in a gap between states, whereas the E F in metals lies in the middle of a band of electronic states. For decades, how an insulator is transformed into a metal by manipulating either the E F or the states has been one of the central themes in condensed matter physics [1] , [2] , [3] , [4] , whatever it is a band or Mott insulator. The current strategies in making such a transition in materials, whether in form of bulk or thin film, can be summarized mainly in three aspects: (1) chemical doping either shifts the E F towards the conduction band (CB)/valence band owing to the infusion of carriers, or modulates gaps by altering electronic structures [5] , [6] , (2) substantial decrease of the ratio U/W between on-site Coulomb interaction ( U ) and bandwidth ( W ) may close the Mott gaps and hence render the E F stand in a band, which could be triggered by the atomic-scale substitutions or the application of external parameters, for example, pressure, heat, electric and magnetic field [7] , [8] , (3) impurity-induced structure disorder, such as the spatial fluctuations in electrostatic potential, initiates an Anderson transition even in a system of non-interacting electrons [9] . Definitely, none have supported a seemingly counter-intuitive route: the use of an insulating layer to induce the insulator-to-metal transition, because neither the well-pinned E F is shifted nor the gaps are eliminated. These considerations do not, however, exclude a more 'internal' feasibility that in a non-stoichiometric, Mott superlattice, there are another two relevant factors—notable lattice distortion and strong e – e interplay—that could be affected fundamentally by the additional insulating layers, thereby offering an opportunity to trigger a desired transition. In this study, we report such a case: A-site excess, non-stoichiometric oxides, La 0.5 Sr n +1−0.5 Ti n O 3 n +1 , shows an unprecedented insulator-to-metal transition, which is driven by an intrinsically insulating SrTiO 3 (STO) unit cell. The transition is accompanied by electron localization due to a complex interplay of electrons and phonons, and is unusual as the majority of electrons in the conducting phase are confined to within an atomic layer forming a two-dimensional electron gas (2DEG). To our knowledge, this is the first report on a transition induced by the dimensionality n in a 3 d Ruddlesden-Popper (RP) homologous series, perhaps opening up yet another useful dimension for property control and customization of the technologically important perovskites. The layered RP oxides, A n +1 B n O 3 n +1 (see Supplementary Fig. S1 ), owing to the richness in their inherent properties [10] , are continuing to be of intense interest in both the fundamental physics and technological applications. This interest is further aroused by the rising possibility in incorporating function-providing elements (A′) into the RP faults (A′ x A n +1− x B n O 3 n +1 ) and in manipulating the dopants at the atomic scale, thereby bringing novel performances to electronics [11] , [12] . Materials preparation and characterization The oxide series we considered, La 0.5 Sr n +1−0.5 Ti n O 3 n +1 , is a class of multifunctional compounds, which displays in structure the sequence of one rock-salt La 0.5 Sr 0.5 O layer intercalated between n blocks of perovskite STO (ref. 13 ) ( Fig. 1a ). 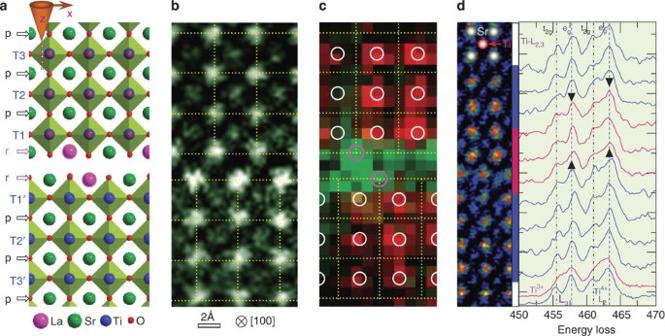Figure 1: Atomic-resolution imaging of the La0.5Sr5.5Ti5O16structures using the STEM and EELS. (a) Crystal structure of the layered RP perovskite, La0.5Sr5.5Ti5O16, viewed from [100] direction. Note that the upper and lower portion has been omitted and that the A-sites consist of 9-coordinated r (at fault) and 12-coordinated p-sites (in the perovskite layers). (b) HAADF-STEM image of the RP observed from the [100] direction. (c) Core-loss image of the combined Ti-L2,3(red) and La-M4,5(green) edges. The white and pink circles indicate positions of Ti and La columns, respectively. (d) HAADF image (left) and Ti-L2,3edge EELS profile (right) recorded across the RP fault. The spectra of Ti3+and Ti4+are given at the bottom as a reference, which are obtained from thick area of LaTiO3and STO (close to bulk). Figure 1: Atomic-resolution imaging of the La 0.5 Sr 5.5 Ti 5 O 16 structures using the STEM and EELS. ( a ) Crystal structure of the layered RP perovskite, La 0.5 Sr 5.5 Ti 5 O 16 , viewed from [100] direction. Note that the upper and lower portion has been omitted and that the A-sites consist of 9-coordinated r (at fault) and 12-coordinated p-sites (in the perovskite layers). ( b ) HAADF-STEM image of the RP observed from the [100] direction. ( c ) Core-loss image of the combined Ti-L 2,3 (red) and La-M 4,5 (green) edges. The white and pink circles indicate positions of Ti and La columns, respectively. ( d ) HAADF image (left) and Ti-L 2,3 edge EELS profile (right) recorded across the RP fault. The spectra of Ti 3+ and Ti 4+ are given at the bottom as a reference, which are obtained from thick area of LaTiO 3 and STO (close to bulk). Full size image The thin films of La 0.5 Sr n +1−0.5 Ti n O 3 n +1 ( n =2–5) superlattice were grown using the pulsed laser deposition (PLD) method combined with a repeated temperature modulation technique [14] , which allows an independent deposition of SrO (La 0.5 Sr 0.5 O) layers and STO blocks at their own pre-optimized temperatures. With this approach and the optimized growth parameters, the crystallinity of the deposited films was found to be improved significantly [15] . Figure 1b shows a representative image of the RP phase with n =5 taken with a spherical-aberration-corrected high-angle annular dark-field scanning transmission electron microscope (HAADF-STEM). As the intensity of an atomic column in this imaging mode is, to a good approximation, directly proportional to the square of atomic number (Z) (ref. 16 ), brighter spots in the image represent columns of Sr, whereas darker ones indicate columns of Ti. Evidently, there appears a (½ a , ½ a ) shift ( a : in-plane lattice constant) between the ( n +½)-unit-cell-thick perovskite slabs in the basal plane, which means a successful output of the RP structure. However, columns of La and O are not scattered strongly enough to be visualized owing to the partial occupation of La at the A-sites and to the small Z of O. To determine the La sites quantitatively, we performed an atomic-resolution electron energy-loss spectroscopy (EELS) analysis [17] on the La-M 4,5 edge together with the Ti-L 2,3 edge as a reference ( Fig. 1c ). The smaller circles in the core-loss image ( Fig. 1b ) correspond correctly to the Ti columns, thus providing a direct evidence that the La (larger circles) diffuses into the both r sites (9-coordinated and located within the rock-salt layers), although they are originally deposited at one r-site only. This r-site-ordered, stripped-off La 3+ ion introduces an additional electron that resides mainly on the Ti 3 d orbitals, inferring that the Ti ions nearest to the fault are of a mixed valence state of +3/+4. This is confirmed by the EELS spectra of Ti-L 2,3 edge ( Fig. 1d ), showing a broader profile (marked with arrows) for the Ti layers neighbouring the fault. Furthermore, this implies the formation of 2DEG in the La 0.5 Sr 5.5 Ti 5 O 16 [18] (for reference, L 2,3 edges of Ti 3+ and Ti 4+ in their corresponding bulks, LaTiO 3 and STO, are presented at the bottom of Fig. 1d ). 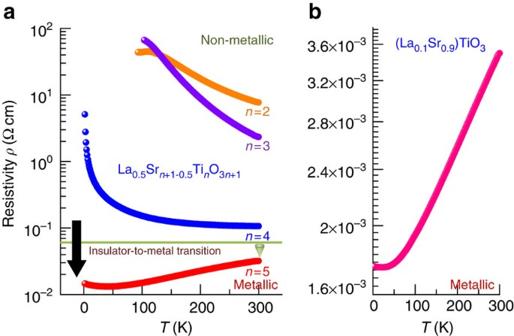Figure 2: TemperatureTdependence of resistivityρ. (a) Resistivity as a function of temperature for the La0.5Srn+1−0.5TinO3n+1(n=2–5) thin films showing clearly the insulator-to-metal transition asnis beyond the threshold. (b) Temperature dependence ofρfor the thin film of La0.1Sr0.9TiO3perovskite. Conductivity measurements Figure 2a presents resistivity ρ as a function of temperature T for the films, where a transition from the insulating ground state ( ρ increases with decrease of T ) to metallicity maintained down to 20 K is discovered, as the n goes beyond 4. This is rather unexpected because the carrier density, a critical driving force to launch a transition, is in fact constant for all the RP films (1.4×10 21 cm −3 ), as evaluated nominally from the concentration of the carrier-providing La atoms. In addition, the transition is induced by the insulating units, which are conventionally believed to produce no metallic states at all for an insulator and even impair a conducting nature for a metallic superlattice. The RP films with n no more than 4 are of insulating nature, in stark contrast to the metallicity shown in their ending member ( Fig. 2b ) (ref. 19 ), which implies that their carrier transport states are susceptible to be spatially localized. This scenario is further supported qualitatively by a Hall measurement on the film with n =5, showing that its carrier concentration at T =300 K reaches a value as low as 2.8×10 20 cm −3 (see the arrow in Fig. 2a ), merely one-fifth of what one expects from the nominal La concentration (the carrier concentrations for the films with n =2–4 are not measurable owing to their high resistivity). Figure 2: Temperature T dependence of resistivity ρ . ( a ) Resistivity as a function of temperature for the La 0.5 Sr n +1−0.5 Ti n O 3 n +1 ( n =2–5) thin films showing clearly the insulator-to-metal transition as n is beyond the threshold. ( b ) Temperature dependence of ρ for the thin film of La 0.1 Sr 0.9 TiO 3 perovskite. Full size image First-principles calculations on energetics and electronic structures To gain more insights into the physical mechanism of the transition and the quantum nature of the conducting states, we have performed a comprehensive density-functional-theory (DFT) calculation using the generalized gradient approximation functional plus the one-site repulsion U -method. We first determine the La occupation at the A-sites by calculating the formation energy of Sr substitution by La ( E f (La Sr )) using the relation [20] where the E tot (defect) and E tot (host) are total energies of the supercell with and without the point defects, and n i and μ i are the number and chemical potential of the i atom ( i =La, Sr), respectively. The energy calculations indicate that La atoms prefer segregating at the r-sites to the p-sites (12-coordinated and located within the perovskite layers) by saving at least 0.13 eV in E f , which supports the observed r-site ordering of La ( Fig. 1c ). Among all the likely positions examined, the combined sites, A and C (labelled in Fig. 3a ), turn out to have the lowest E f , meaning that they are the most energetically stable occupations for La, in a good agreement with the above EELS mapping ( Fig. 1c ). 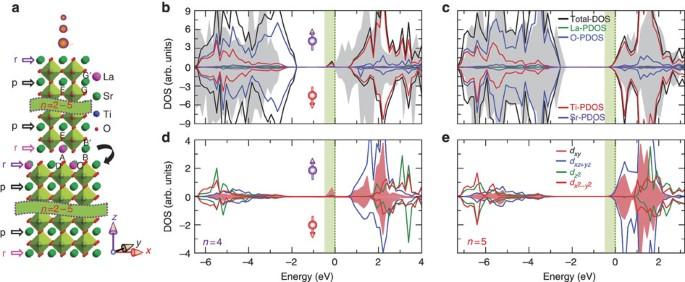Figure 3: Predicted transition from insulator to metal in the RP series. (a) A ball-model view of a periodicity of the RP phase. The substitutional sites we considered for La in A-sites are labelled A–G according to the structural symmetry. (b) Total DOS and partial DOS (PDOS) plots of the La, Ti, Sr and O atom contributions for the relaxed RP structure withnof 4 (insulator) and (c) those withnof 5 (metal). The total DOSs for their corresponding ideal, unrelaxed RP structures are given as well in grey background. (d) PDOS plots of the Ti-3dorbitals for the relaxed RP phase withnof 4 and (e) those withnof 5, where the PDOSs for the Ti-dxyorbital are highlighted by shading. Note that the DOSs for the RP phases withnof 2 and 3 are similar to those withn=4 (Supplementary Fig. S2) and that this analogy is also observed between the cases ofn=5 and 6. Figure 3b–e presents the electronic structures of the RP series, calculated using the energetically stable atomic geometries. Surprisingly, our calculations unambiguously reproduce the insulator-to-metal transition as n passes through the threshold value, 4: below this threshold, the overall features of density of states (DOS) around E F for the superlattices are similar (see also Supplementary Fig. S2 ), with E F lying in the gap splitting the filled spin-up Ti- d xy orbital (lower Hubbard band) from the rest of unfilled d levels (upper Hubbard band); above the threshold, the E F shifts upward by ∼ 1.1 eV and ultimately overlaps the tails of the Ti- t 2g bands for both spins, meaning a full metallicity. This predicted transition is further verified by performing calculations using different supercell sizes, and the metallic state is found to emerge in the case of n =6 as well. Figure 3: Predicted transition from insulator to metal in the RP series. ( a ) A ball-model view of a periodicity of the RP phase. The substitutional sites we considered for La in A-sites are labelled A–G according to the structural symmetry. ( b ) Total DOS and partial DOS (PDOS) plots of the La, Ti, Sr and O atom contributions for the relaxed RP structure with n of 4 (insulator) and ( c ) those with n of 5 (metal). The total DOSs for their corresponding ideal, unrelaxed RP structures are given as well in grey background. ( d ) PDOS plots of the Ti-3 d orbitals for the relaxed RP phase with n of 4 and ( e ) those with n of 5, where the PDOSs for the Ti- d xy orbital are highlighted by shading. Note that the DOSs for the RP phases with n of 2 and 3 are similar to those with n =4 ( Supplementary Fig. S2 ) and that this analogy is also observed between the cases of n =5 and 6. Full size image A Jahn-Teller (JT) effect turns up in the RP phases with the n of no more than the threshold, as the occupied Ti- d xy states are lowered substantially, splitting the 3 d levels [21] (see Fig. 3b and in the Supplementary Methods ). In general, the presence of a JT distortion can be viewed as an empirical litmus test for the localized electronic states. 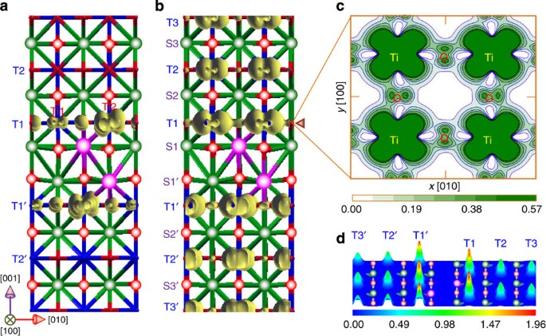Figure 4: Charge variation accompanied with the transition. (a) Isosurface along the (100) plane, integrated in the energy window (EF−0.5 eV,EF) for the RP phase withn=4 and (b) that withn=5, suggesting a change of electronic states from localized to itinerant. The largest to smallest balls represent the La, Sr and O atoms, respectively. (c) Charge contours of occupied states in the conduction bands plotted on the (001) plane for the TiO2layer nearest to the fault of the RP phase withn=5. (d) Density of electrons occupying different perovskite layers of the conducting RP phase as a function of distance from the fault, showing the confinement of carriers to the TiO2layers proximal to the fault. Figure 4a illustrates an electron-density plot for the filled states in the case of n =4, where charges are indeed localized to within two TiO 2 layers closest to the fault in a two-dimensional manner. This agrees well with the two remarkably lowered bands in the band-structure plot, and is further verified by the non-equilibrium quantum transport calculations ( Supplementary Fig. S3 ) [22] , [23] , showing a small transmission coefficient at E F . Structurally, the creation and stabilization of the localized states are associated with the spontaneous lattice distortions (versus bulk), which are characterized by a substantial length imbalance for the La–Ti bonds ( ∼ 0.04 Å), accompanied by a considerable increase in distance between Ti1 (Ti2) and apical O ions ( ∼ 0.05 Å) and by a decrease (increase) of the in-plane Ti1–O (Ti2–O) distances ∼ 0.05 Å ( ∼ 0.04 Å) ( Supplementary Fig. S4 ). This structural shift of Ti ligand O from the Oh to C 2v breaks the crystal symmetry, which could stabilize the largely split orbitals in the non-conducting RP phases. As a consequence, electronic overlap of the 3 d -2 p -3 d orbitals is locally weakened for the conductance-channel network, Ti-O-Ti, which lowers significantly the W and hence produces a gap opening [24] . Further evidence for the role of lattice distortion in the electron localization comes from the calculations on electronic structures of the structurally perfect (unrelaxed) RP phases, that is, the artificially undistorted cases. The results reveal that the CB is shifted by more than 0.8 eV closer to E F and is eventually occupied partially (grey shading in Fig. 3b ). These do not, however, destabilize an alternative mechanism that may cause the electron localization, namely, the e – e correlations, since Mott's landmark work [25] . In contrast, its importance is supported by our DFT calculations without U , which indicate metallicity for the RP with n of no more than the threshold. We therefore conclude that the insulating states result from a complex interplay between the electron–lattice coupling and the e – e correlations. Figure 4: Charge variation accompanied with the transition. ( a ) Isosurface along the (100) plane, integrated in the energy window ( E F −0.5 eV, E F ) for the RP phase with n =4 and ( b ) that with n =5, suggesting a change of electronic states from localized to itinerant. The largest to smallest balls represent the La, Sr and O atoms, respectively. ( c ) Charge contours of occupied states in the conduction bands plotted on the (001) plane for the TiO 2 layer nearest to the fault of the RP phase with n =5. ( d ) Density of electrons occupying different perovskite layers of the conducting RP phase as a function of distance from the fault, showing the confinement of carriers to the TiO 2 layers proximal to the fault. Full size image Similar sizable distortions are not present in the RP with n beyond the threshold (<0.01 Å), which electronically results in broadly distributed charges in a three-dimensional manner ( Fig. 4b ). As the electron density of Ti(3 d ) bands in this system is far from half filling, the correlation effects are not expected to alter the metallic states fundamentally, as confirmed further by our calculations without U , showing the overlap of E F with the tail of Ti( d ) t 2g states (shading in Fig. 3c ). These imply such a mechanism: although the intercalation of insulating unit itself provides no current-carrying states at all, it might switch locally (around the faults) the Ti valence from +3 towards +4, and in the meanwhile eliminate the lattice polarization between the RP faults. Both are crucial to induce a transition in such an A-site-excess, Mott-insulating superlattice. It is noteworthy that an atom-by-atom examination on d occupancy of each Ti in the insulating phases reveals that both the overall feature and bader charge of the Ti nearest to the fault approach those of Ti in bulk LaTiO 3 , thereby validating the understanding of insulating nature from the Mott mechanism. As the n passes through the threshold, the relieved lattice distortion and e – e correlation push the largely split d xy bands and E F upward the CB, which results in a 'leakage' of the localized electrons (Ti- d 1 -like electronic wavefunction) out of the T1 and T1′ layers ( Fig. 4a ) and ultimately into the inner Ti layers of STO block ( Fig. 4b ). Furthermore, the lattice reconstruction has also relevant consequences for electronic physics, leading, in particular, to a novel planar xy orbital ordering in a butterfly shape ( Fig. 4c ). In addition, we observe that (1) charges on the T1 and T1′ layers in the case of n =5 are spatially connected owing to the hybridization of Ti- d orbital with O- p level, and (2) charges are confined, to a large extent, in the two layers nearest to the fault ( Fig. 4d ), which is due to the low potential there ( Supplementary Fig. S5 ), as in the case of the (SrTiO 3 ) n /(LaTiO 3 ) 1 superlattice showing a wedge-shaped potential well close to the La layer [26] . These heavily confined electrons reduce the Ti in the T1 (T1′) layer from Ti 4+ towards Ti 3+ , which explains the broadened EELS profiles in the Ti-L 2,3 edge ( Fig. 1d ). 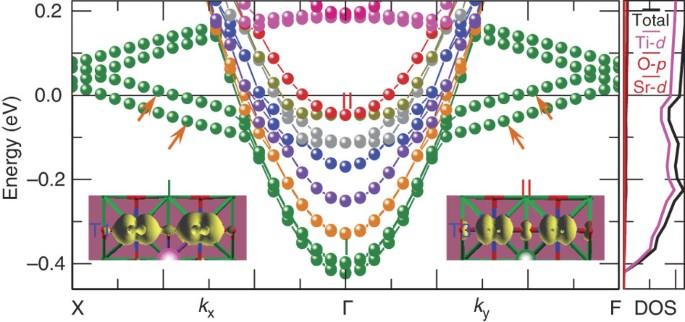Figure 5: Band structure nearEFdemonstrating the formation of 2DEG in the conducting RP phase. Left panel: conduction band dispersions shown along thexyplane withX=π/a(1,0,0) andF=π/a(0,1,0), where the 'a' is in-plane lattice constant. The parabola-like dispersion of conduction bands implies that free electron is a good starting approximation to examine behaviours of the 2DEG. The isosurface of the T1 layer corresponding to the lowest band I is presented in left inset and that of the T3 layer corresponding to the band II is shown in right inset. Right panel: total DOS and its respective atomic contributions: Ti-d, O-pand Sr-dorbitals, showing that the conduction bands are predominantly of Ti(d) nature. TheEFposition is aligned to zero. Both the charge contour and EELS analyses strongly suggest the formation of 2DEG in the conducting RP, which is further corroborated in the band structure shown in Figure 5 . The occupied CBs, which are made mainly out of Ti( d ) t 2g states (right panel), exhibit a nearly quadratic dispersion, except two lowest bands having a flat dispersion in the k -space away from Γ point (marked by arrows). This phenomenon can be attributed to the orbital difference between the two bands and the remainder of occupied CBs, possibly owing to the crystal field. These two unusual bands, which correspond mainly to the two TiO 2 layers closest to the fault, demonstrate again the presence of 2DEG in the conducting RP. However, in the cases of non-conducting RP, the lowest CBs sit far above E F owing to the split of the two d xy bands ( Fig. 3d ) and are therefore fully unoccupied. As indicated from the electron wavefunctions in left inset, the states for such two bands (type I) are indeed confined spatially onto the T1 (T1′) layer in a d xy -like manner because of the large hopping matrix elements for the d xy orbitals along x and y directions. As two-dimensional states are prone to either be Anderson localized by disorder or form self-trapped polarons by a JT coupling, they contribute less to electron transport (recall the orbital ordering). On the other hand, there exists an alternative class of electrons (type II), which originate from the shallower Ti( xy ) bands yet spread inward over several Ti layers (right inset) [27] . By fitting the band to a parabola, E ( k )=|ħ k | 2 /(2 m *)+ b , we find that these electrons have smaller effective masses ( m *) with accordingly higher mobilities along the fault plane in comparison with the type I electrons, which are difficult to localize and would therefore contribute to the transport. On this basis, the low carrier density observed in the Hall measurement could be explained by the likely trapping of type I electrons leaving a lower density of higher mobility type II electrons. Figure 5: Band structure near E F demonstrating the formation of 2DEG in the conducting RP phase. Left panel: conduction band dispersions shown along the xy plane with X = π / a (1,0,0) and F = π / a (0,1,0), where the ' a ' is in-plane lattice constant. The parabola-like dispersion of conduction bands implies that free electron is a good starting approximation to examine behaviours of the 2DEG. The isosurface of the T1 layer corresponding to the lowest band I is presented in left inset and that of the T3 layer corresponding to the band II is shown in right inset. Right panel: total DOS and its respective atomic contributions: Ti- d , O- p and Sr- d orbitals, showing that the conduction bands are predominantly of Ti( d ) nature. The E F position is aligned to zero. Full size image This remarkable transition is unlikely to be a coincidence, especially considering the recent evidence that the structural distortion and correlation effect are even important in inducing a transition in the 4 d and 5 d transition metal oxides [28] , [29] . As the 3 d orbitals are spatially less extended plus much smaller (larger) W ( U ) values [7] , the presence of metallic states driven from the well insulating ground states by an insulating unit in a controllable way is quite unique. Rather, it is also applicable to a series of RP phases with distinct A′, of which the RP phases with another two types of carrier-providing elements, Y 3+ and Nd 3+ , have also been suggested through our extensive calculations to undergo a similar transition. Keeping in mind the critical role of the SrTiO 3 in the fascinating oxide-based electronics, the ability to precisely tailor the intrinsic properties of its derivatives adds new practical routes for the design of sophisticated devices in this field. Sample growth and microscopic characterization Thin films were prepared by the PLD with a KrF excimer laser (248 nm, 2 Hz, and 1.5 J cm −2 ) in a high vacuum chamber with the oxygen pressure of 10 −6 torr. Single STO crystals and pellets of La 0.5 Sr 0.5 O were applied as target materials and the atomically flat, TiO 2 -terminated (001) STO as substrates. Growth temperatures of STO and La 0.5 Sr 0.5 O were controlled at 848 and 1,053 K, respectively, using a semiconductor laser heating system. During the growth, the intensity oscillations of reflection high-energy electron diffraction patterns were monitored in situ to precisely control the layer thickness on an atomic level. The deposited films were estimated as thick as 90 nm. After the growth, all films were annealed at 673 K in air for 1 h to refill residual oxygen vacancies. Specimens for STEM observations were prepared by cutting, mechanically grinding, and dimpling the deposited samples down to about 20 μm. In the Ar ion-beam thinning processes, we used accelerating voltages of 2–4 kV and an incident beam angle of 6° to avoid radiation damage. The HAADF images were observed using a 200 kV STEM (JEM-2100F, JEOL) equipped with an aberration corrector (CEOS Gmbh), which offers an unprecedented opportunity to probe structures with a sub-Å resolution. A HAADF detector with an inner semi-angle of over 60 mrad was used. The EELS was recorded using a Gatan Enfina system equipped on the STEM with a energy resolution at full width of half maximum of 1.6 eV. The electrical conductivity was measured using a physical property measurement system (Quantum Design) for the temperatures ranging between 300 and 2 K, and a diluted refrigerator from 2 K to 70 mK. Calculational methodology Calculations of energies and electronic structures were performed using the VASP code within the DFT [30] . We applied the projector augmented wave approach with a 4 × 4 × 1 k -point grid and a cutoff energy of 400 eV. The generalized gradient approximation plus U -method was used with U =5 and J= 0.64 eV for the Ti- d states, and U f =11 and J f =0.68 eV for the La f states. We further tested different U -and J -values [31] and found that they affect neither the transition nor the critical threshold value fundamentally. In addition, the above parameters were confirmed to enable an accurate prediction of both atomic and electronic structures of this system. The RP phases were modelled by a 2 × 2 supercell along transverse directions and further by a doubled supercell to examine the size effect. All atoms in the supercells were fully relaxed till the magnitude of force on each atom fell <0.05 eV Å −1 . Electron transport were calculated using the state-of-the-art quantum transport technique, that is, the fully self-consistent non-equilibrium Green's function method combined with the DFT [22] , which was implemented in the Atomistix Toolkit code [23] . The model used for calculating the transport can be schematically divided into the left semi-infinite electrode, scattering region and the right semi-infinite electrode ( Supplementary Fig. S3 ). The total energy was well converged to within 1–2 meV per atom upon using 2 × 2 k -points and a cutoff of 100 Ry. A 10 × 10 k -point mesh was then used to obtain converged transmission spectra. Stoichiometry in the fabricated RP phases Spectroscopic studies and theoretical calculations demonstrate that neither unwanted dopants nor oxygen vacancies are detected in the films and that the oxygen deficiency, if there is, would not affect the transition fundamentally. These therefore ensure that all the films discussed here are structurally stoichiometric in their RP forms, so that the varying transport behaviours can be reasonably understood on a purely electronic mechanism. First, we applied an extremely clean and ultrahigh vacuum PLD deposition system to fabricate the La-doped RP series. In addition, the chemical reagents used to prepare the targets had purity as high as 4 N or more and the films were prepared carefully to avoid contamination, which ensured that the unwanted impurity incorporation was minimized to our best. This is also supported by our further EELS and energy-dispersive X-ray spectroscopy analyses, showing that there appear La, Sr, Ti and O elements only without any identifiable impurity in the samples within our detection capability. To eliminate the possible conduction arising from the residual oxygen vacancies, we have annealed all the samples very carefully, as aforementioned, which has produced insulating behaviours for the undoped RP phases with n ranging from 2 to 5, as well as for the homo-epitaxial STO films (conductivity is zero under the inspection using the conventional measurement setup), as described in our previous report [15] . We have also had taken the EELS spectra of each atomic layer with a probe size <0.7 Å. The spectroscopic chemical mapping of the oxygen O-K edge reveals that oxygen is present universally in the sample with no significant depression in the layers around the fault ( Fig. 6b ). In addition, the O-K edge profiles acquired from the La-doped region matches well with that from the STO block region ( Fig. 6c ), suggesting that the oxygen occupancy does not alter abruptly when approaching the fault. This is further confirmed through a layer-by-layer analysis of the EELS spectra of O-K edges ( Fig. 7 ) showing that the profiles of the O layers in the superlattice resemble, to a large extent, that of the O in a single crystalline STO bulk, whatever the O comes from the fault or block region. 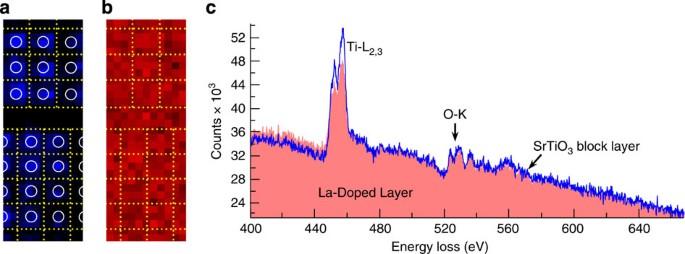Figure 6: Compositonal characterization using STEM-EELS. An atomic-resolution chemical map of the RP phase withn=5 showing (a) Ti-L2,3and (b) O-K edge spectroscopic signals. The circles inadesignate the sites of Ti. (c) Electron energy loss spectrum obtained from both the STO block layer and the region around La-doped layer suggesting a similarity between them in overall feature of the O-K edge. Figure 6: Compositonal characterization using STEM-EELS. An atomic-resolution chemical map of the RP phase with n =5 showing ( a ) Ti-L 2,3 and ( b ) O-K edge spectroscopic signals. The circles in a designate the sites of Ti. ( c ) Electron energy loss spectrum obtained from both the STO block layer and the region around La-doped layer suggesting a similarity between them in overall feature of the O-K edge. 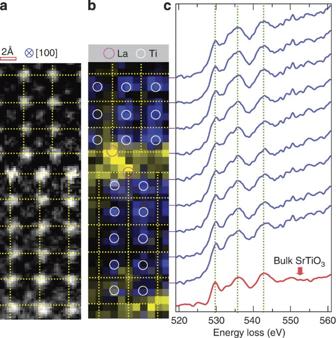Figure 7: Layer-by-layer analysis using STEM and EELS. (a) HAADF-STEM image of the RP withn=5 observed from the [100] direction. (b) Core-loss image of combined Ti-L2,3(blue) and La-M4,5(yellow) edges. (c) The background corrected EELS profile of the O-K edges recorded across the fault. The spectrum of O in a single crystalline STO bulk is given as well for a reference. Full size image Figure 7: Layer-by-layer analysis using STEM and EELS. ( a ) HAADF-STEM image of the RP with n =5 observed from the [100] direction. ( b ) Core-loss image of combined Ti-L 2,3 (blue) and La-M 4,5 (yellow) edges. ( c ) The background corrected EELS profile of the O-K edges recorded across the fault. The spectrum of O in a single crystalline STO bulk is given as well for a reference. Full size image Theoretically, we introduced an O vacancy into the La-doped RP phase with n =5 at a variety of possible sites and calculated total energy of each relaxed system, as listed in Supplementary Table S1 . Interestingly, we find that O vacancy prefers segregating at the SrO layer to the TiO 2 layer. More importantly, O vacancy is much more favourable to rest at the central SrO layer of the STO block than at the SrO layer nearest to the fault by saving at least 0.62 eV in total energy ( Supplementary Table S1 ). This preference is also applicable to the undoped RP systems showing that the energy for an O vacancy at the central SrO layer of the STO block is lower than that at the SrO layer proximal to the fault by 0.72 eV. It is worthy of mentioning that this preference of O vacancy at central SrO layer of the STO block is also confirmed in the RP phase with n =4 after the introduction of O vacancy. As an O vacancy introduces additional electrons into its host system, valence of Ti in the TiO 2 layer nearest the central SrO layer of the STO block should be affected severely. However, such an influence is seen only for the Ti in the TiO 2 layers nearest to the fault from the EELS profile of Ti-L 2,3 edge ( Fig. 1d ), suggesting strongly stoichiometry of the RP phases. Furthermore, these indicate that the formation of 2DEG surrounding the fault in the conducting RP should not be attributed simply to the O vacancy, but arise from the doped La at the fault. In this sense, the combined spectroscopic analyses with theoretical calculations imply that the origin of the observed different transport properties should not be understood from the structural non-stoichiometry in their RP phases, but from the purely electronic mechanism. How to cite this article: Wang, Z. et al . Dimensionality-driven insulator–metal transition in A-site excess non-stoichiometric perovskites. Nat. Commun. 1:106 doi: 10.1038/ncomms1111 (2010).